A fast and low-power microelectromechanical system-based non-volatile memory device Several new generation memory devices have been developed to overcome the low performance of conventional silicon-based flash memory. In this study, we demonstrate a novel non-volatile memory design based on the electromechanical motion of a cantilever to provide fast charging and discharging of a floating-gate electrode. The operation is demonstrated by using an electromechanical metal cantilever to charge a floating gate that controls the charge transport through a carbon nanotube field-effect transistor. The set and reset currents are unchanged after more than 11 h constant operation. Over 500 repeated programming and erasing cycles were demonstrated under atmospheric conditions at room temperature without degradation. Multinary bit programming can be achieved by varying the voltage on the cantilever. The operation speed of the device is faster than a conventional flash memory and the power consumption is lower than other memory devices. As the first demonstration of a non-volatile semiconductor memory with a floating gate was introduced in the mid-1960s [1] , various types of memory devices, such as PROM, EPROM, EEPROM [2] and flash memory [3] have been developed. At present, NAND- and NOR-type flash memories are widely used for computer memories and other portable devices because of the low cost of production and well-developed fabrication technology. However, a flash memory has a relatively low operation speed with ∼ 10 μs programming and ∼ 10 ms erasing time, much slower than other electronic components [4] , [5] . Recently, extensive studies have been performed to improve memory performance in terms of retention time, endurance, integration, speed and energy consumption. Non-volatile data storage devices, such as FERAM [6] , MRAM [7] , PRAM [8] , SONOS [4] , [9] and ReRAM [10] , [11] , [12] , have been investigated. The demonstration of carbon nanotube (CNT) field-effect transistors (FET) [13] , [14] has opened up the possibility of using CNT in non-volatile memory devices. However, to date, any demonstrated devices, based on static CNT transistors, have limitations of low operation speed [15] , [16] , [17] and/or short retention times [18] , [19] . Such limitations may be overcome by making use of mechanical motion. Radio frequency microelectromechanical system (RF MEMS) switches have been shown to provide several advantages such as high-speed switching, ultra-low losses, high isolation, high linearity of relays and low-power consumption [20] . Memory devices based on the electromechanical motion of nanotubes have been demonstrated, including three terminal relays [21] , crossed nanotube arrays [22] and vertical nanoscale memory cells [23] ; however, there are considerable challenges associated with the reproducible fabrication and operation of such devices. In this article, we demonstrate a novel non-volatile memory device consisting of a static transistor channel and a movable cantilever switch that is used to directly charge/discharge a floating gate. A CNT is used as the active channel between the source and drain electrodes, and the amount of charge on the floating gate is controlled by the cantilever. The basic memory properties of our device, such as the retention characteristics at the programmed/erased states and the endurance performance, are investigated. The possibility of multinary bit programming with the device was demonstrated by changing the voltage on the cantilever. The write and the erase operation speed were estimated by measuring the switching speed of the cantilever. The power consumption of the device was calculated and compared with commercially available flash memories. The experimental results show that the device performance is superior to that of conventional flash memories. Device fabrication and operation concept The design concept can easily be extended to other memory architectures in which a floating gate needs to be quickly and efficiently charged and discharged, however, there is an advantage of the CNT-FET design as demonstrated here. The floating gate provides a potential barrier for the charge carriers in the CNT-FET and can rapidly switch between on and off states [24] . 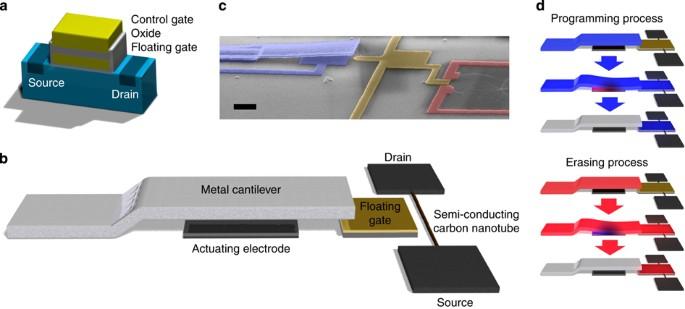Figure 1: Device concept and operation processes. (a) Schematic illustration of an ordinary flash memory cell. A floating gate surrounded by an insulating layer is located on the MOSFET. Electrons are injected/tunnel through the thin oxide layer and are stored in the floating gate. (b) Schematic diagram of the MEMS-based non-volatile memory device. The CNT is used for the source/drain channel and a MEM cantilever is added to transfer charges to the floating gate. (c) Field-emission scanning electron microscope image of the device. Colour-coded to show the main elements: source/drain (red), floating gate (yellow) and cantilever/actuating electrode (blue). Scale bar, 2 μm. (d) Diagrams demonstrating the programming (upper three panels)/erasing (lower three panels) processes. Blue/red colours indicate the polarities± of the applied voltages. In ordinary flash memories, the floating gate, surrounded by a thin insulating barrier, is placed on a metal–oxide–semiconductor field-effect transistor (MOSFET) channel [1] as shown in Figure 1a . Electrons tunnel to the floating gate through the insulating dielectric on application of a high voltage to the control gate. The tunnelling of electrons through the oxide layer causes a time delay resulting in a low operation speed and also limits the number of useful cycles that can be achieved. To greatly increase the operation speed, we use a microelectromechanical (MEM) metallic cantilever that directly contacts a metallic floating gate. A schematic drawing of the device is illustrated in Figure 1b . Unlike a conventional flash cell, the channel between source and drain in our device is replaced with a semiconducting CNT, and a MEM cantilever and actuating electrode are introduced. The cantilever is anchored at one end and it is suspended above the actuating electrode and the floating gate. When a bias voltage is applied to the actuating electrode, the resultant electrostatic force pulls down the cantilever until it contacts the floating gate. The cantilever is composed of Cr/Al/Cr triple layers and the floating gate is made of Au. The Au floating gate is placed on top of an 80-nm-thick Al 2 O 3 layer. In this configuration, the floating gate is charged at the instant of contact. The charge on the floating gate controls the source-drain current through the CNT channel. No back gate voltage is applied. Devices with both side floating gates and top floating gates were fabricated and characterized. A field-emission scanning electron microscope image of the whole structure is shown in Figure 1c . The source/drain, floating gate and cantilever/actuating electrode are coloured by red, yellow and blue, respectively. The detailed fabrication process is described in the Methods section and the Supplementary Figures S1 and S2 . The CNTs used in our experiment were p-type semiconducting. The on/off switching ratio was determined to be 10 4 –10 5 by measuring the back gate voltage dependence of the source-drain current of the CNT channel (see the Supplementary Fig. S3 ). The operation of the device is shown in Figure 1d . Here the red and blue colours indicate positive and negative polarities, respectively. The programming process is the following (see Fig. 1d , upper): (1) when a positive voltage is applied to the actuating electrode while the cantilever is biased negatively, the cantilever is pulled down by the attractive electrostatic force to the floating gate. (2) At the moment of contact, the negative charges in the cantilever charge the floating gate instantaneously. By inducing negative charges on the floating gate, the CNT channel is turned 'ON' with hole-transport. We define this as the 'programmed state' or bit '1'. (3) By turning off the actuating electrode voltage, the cantilever is moved back to the original position and the contact between the cantilever and the floating gate is switched off. The floating gate remains negatively charged, and the CNT channel is maintained in the 'programmed state'. The 'erased state' or bit '0' is obtained by reversing the programming processes ( Fig. 1d , lower). (The continuous on–off switching processes are shown in the Supplementary Video .) Figure 1: Device concept and operation processes. ( a ) Schematic illustration of an ordinary flash memory cell. A floating gate surrounded by an insulating layer is located on the MOSFET. Electrons are injected/tunnel through the thin oxide layer and are stored in the floating gate. ( b ) Schematic diagram of the MEMS-based non-volatile memory device. The CNT is used for the source/drain channel and a MEM cantilever is added to transfer charges to the floating gate. ( c ) Field-emission scanning electron microscope image of the device. Colour-coded to show the main elements: source/drain (red), floating gate (yellow) and cantilever/actuating electrode (blue). Scale bar, 2 μm. ( d ) Diagrams demonstrating the programming (upper three panels)/erasing (lower three panels) processes. Blue/red colours indicate the polarities± of the applied voltages. Full size image Retention characteristics To investigate the non-volatility of the device, the retention times of programmed/erased states were measured. 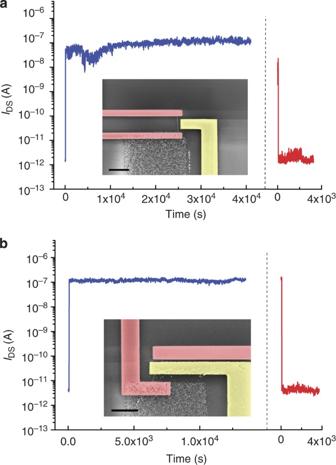Figure 2: Electrical characterizations of CNT memory devices. (a,b) Retention times for the programmed (negative cantilever bias, blue line)/erased (positive cantilever bias, red line) states were monitored in the side-floating gate (a) and top-floating gate (b) devices. TheIDSpersisted without any significant degradation. Insets in theaand thebshow the colour-coded FE-SEM images of the measured devices. Red and yellow colours indicate the source/drain and floating gate, respectively. Scale bars, 1 μm. Figure 2a shows retention characteristics for a side-floating gate device. The device was initially erased by applying +4 V on the cantilever and pulsing (200 ms pulse duration) −12 V on the actuating electrode. The programmed state was obtained by applying −6 V on the cantilever and pulsing (200 ms pulse duration) +10 V on the bottom electrode. The source-drain current ( I DS ) of the CNT-FET in the programmed state (blue line) was monitored with V ds =100 mV for 41,000 s (more than 11 h). After the retention test of the programmed state, the erased state was also monitored (red line). Figure 2b shows similar retention characteristics of a top-floating gate device, where 24 V was applied between the cantilever and the actuating electrode. The I DS through the CNT-FET is retained at a constant value in each state with ca 4–5 orders of magnitude difference between off and on states. There is no sign of degradation of this value within the measurement time window (up to 41,000 s), a much longer retention time is expected as the floating gate is completely isolated without any electrical connections or significant leakage once the cantilever has been positioned in the up-state. Figure 2: Electrical characterizations of CNT memory devices. ( a , b ) Retention times for the programmed (negative cantilever bias, blue line)/erased (positive cantilever bias, red line) states were monitored in the side-floating gate ( a ) and top-floating gate ( b ) devices. The I DS persisted without any significant degradation. Insets in the a and the b show the colour-coded FE-SEM images of the measured devices. Red and yellow colours indicate the source/drain and floating gate, respectively. Scale bars, 1 μm. 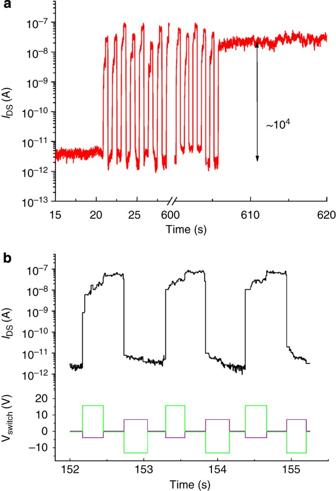Figure 3: Endurance operation. (a) Memory endurance operation under repeated programming/erasing cycles for the side-floating gate device. The test was performed over ca 500 cycles for 600 s withVds=100 mV. (b) Expanded section ofaalso showing the voltages applied to the cantilever (purple line) and activating electrode (green line). Full size image Endurance test Figure 3a shows the endurance characteristics under repeated programming and erasing cycles of a side-floating gate device over 600 s, corresponding to ca 500 cycles. Initially, the device was erased and after 20 s the test was started with the programming and erasing processes as shown in Figure 3a . Figure 3b shows an enlarged section of figure 3a in which the I DS is shown together with the voltage pulses applied to the cantilever (purple) and actuating electrode (green). For the 500 programming and erasing cycles, the device shows successful operation with stable current levels at about 10 −8 A in the programmed state and about 10 −12 A in the erased state. The only limitation in the endurance rate is the number of switching cycles of the MEM cantilever. The typical endurance rate of a flash memory is 10–100 thousand cycles [4] , [5] . On the other hand, MEMS switches are known to have more than 100 million switching cycles [25] , [26] . It can therefore be expected that the CNT memory device presented here can have endurance rates more than 1,000 times better than flash memory devices. Figure 3: Endurance operation. ( a ) Memory endurance operation under repeated programming/erasing cycles for the side-floating gate device. The test was performed over ca 500 cycles for 600 s with V ds =100 mV. ( b ) Expanded section of a also showing the voltages applied to the cantilever (purple line) and activating electrode (green line). Full size image Multinary bit programming The possibility of multinary bit programming for the side-floating gate device has also been investigated. Conventional flash memories have been developed from the single level cell (bit 1 or zero) memory to the multi-level cell by controlling the tunnelling time of electrons through the insulating barrier [27] , [28] . The quantity of charges on the floating gate of the CNT-FET, however, can simply be controlled by adjusting the applied bias voltage to the cantilever and, consequently, the charge level on the gate can affect directly the current flow in the CNT channel. 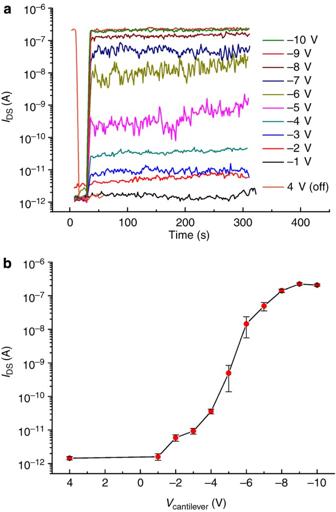Figure 4: Multinary bit programming test for the side-floating gate device. (a)IDScan be controlled by controlling the voltage on the cantilever (−1 V to −10 V with +4 V for erasing). Several programmable states can exist for one device. (b) The averageIDSversusVcantileverderived froma. The error bars indicate the standard deviation of 250 measurement data points for each intermediate state. Figure 4a shows I DS controlled by different cantilever bias voltages. I DS has a value of 10 −12 A when the device is initially in the erased state (+4 V on the cantilever per −12 V of pulse on the actuating electrode). The time duration of the applied pulse on the actuating electrode was fixed at 200 ms for each bit level. The multi-level programmed states are obtained by applying cantilever bias voltages from −1 V to −10 V. At −3 V of bias on the cantilever, the programmed state has ten times higher current (10 −11 A) than that of the erased state (10 −12 A). The current level can be continually increased up to 2×10 −7 A when the cantilever bias voltage has been increased to −9 V. Even though the currents are seen to fluctuate at some intermediate states (for example, at −6, −5 and −2 V of cantilever bias), one can see the clear discrete level of I DS at each programmed state. Retention times for the intermediate programmed states have not been determined but are longer than 300 s. For higher cantilever bias voltages, the current saturates at 2×10 −7 A. The average I DS versus cantilever voltages are plotted in Figure 4b . The error bars indicate the standard deviation of 250 measurement data points during 300 s for each intermediate state. For this memory device, multi-level programming is realized by a simple change of voltage on the cantilever. Therefore, the controllability is much easier and the density of multi-level bits can be much higher than for flash memories. Figure 4: Multinary bit programming test for the side-floating gate device. ( a ) I DS can be controlled by controlling the voltage on the cantilever (−1 V to −10 V with +4 V for erasing). Several programmable states can exist for one device. ( b ) The average I DS versus V cantilever derived from a . The error bars indicate the standard deviation of 250 measurement data points for each intermediate state. Full size image Operation speed Finally, the speed of the presented memory device is much faster than for flash memories, as the programming and erasing operation speeds correspond to the mechanical switching speed of the cantilever. There is no intrinsic time delay due to the tunnelling current as in the flash memory. The spring constant and the resonance frequency of the cantilever are determined by the physical dimensions (width, length and thickness) and Young's modulus of the cantilever material. The maximum speed of the cantilever, in principle given by the resonance frequency, governs the device speed. Measurements were performed to determine the resonant frequency and the switching speed of the cantilevers. The resonant frequency was found to be 8.5 MHz giving a maximum expected switching speed of ca 60 ns. The actual time required to switch the cantilever on was found to be ca 130 ns with ca 145 ns for switching off. The detailed resonance frequency and switching speed measurements on the cantilever are described in the Methods section and the results are shown in the Supplementary Figures S4 and S5 . The switching times are much faster than the speed of conventional flash memories. More systematic investigations on the resonance frequency and switching characteristics are on-going. It would be relatively straightforward to decrease the size of the cantilever to increase the switching speed even more. For example, three terminal relays [21] and vertical memory cells based on actuated individual CNTs have been demonstrated [23] and have switching speeds of at least an order of magnitude higher [29] , although the reproducible fabrication of CNT cantilevers and the problems of stiction at the nanoscale are still challenging. We have developed a memory device consisting of a CNT-FET combined with a metallic MEM cantilever with the following advantages. (1) Endurance rating: for the programming and erasing process in an ordinary flash cell, the thin oxide layer may be damaged by the high electric field needed to transfer electrons, which limits the endurance rating. However, in the device presented here, oxide durability is not an issue as the charges are transferred directly to the floating gate via the metallic cantilever. The endurance rating is determined by the number of switching cycles of the MEM cantilever, and it is known that RF MEMS switches can typically endure approximately three orders of magnitude more cycles than flash memories. (2) Multinary bit programming: the memory device shows well-controlled multi-level programmed states by applying different voltages on the cantilever, thus greatly increasing the density of data storage. (3) Energy consumption: the CNT-FET has low energy consumption, which is comparable to that of conventional MOSFETs [30] and it shows good electrical properties such as high mobility and on/off ratio [31] , [32] . Moreover, the MEMS switch is electrostatically activated and does not consume any current. Therefore, near-zero power is required for each switching operation. The detailed comparison of energy consumption for our device and conventional flash memories is described in Supplementary Discussion . As the presented memory device combines the advantages of both CNT-FET and the MEMS switch, the power consumption is much less than other memories. (4) Operation speed: the speed of the memory device is only limited by the speed of the cantilever switch, so that it is much faster than a flash memory. By replacing the MEMS switch with a NEMS switch, the speed may be further increased by at least an order of magnitude. Device fabrication Highly doped p-type Si wafers with 300-nm-thick oxide grown by low-pressure chemical vapour deposition (CVD) were used in our experiment. On top of this, a matrix of alignment markers with 5 nm Ti per 75 nm Mo and catalyst islands with 10 nm Al 2 O 3 per 0.5 nm Fe were patterned using a Jeol EBX-9300FS electron beam lithography (EBL) machine (Jeol) and deposited by an AVAC HVC600 e-gun evaporator. The CNT growth was carried out for 15 min at 900 °C in a standard thermal CVD process with 1,000 sccm CH 4 /100 sccm H 2 . Source, drain and actuating electrodes were fabricated by depositing 0.5 nm Ti/39.5 nm Pd/50 nm Al 2 O 3 ( Supplementary Fig. S1a ). The oxide layer is required to avoid electrical contact between the cantilever and the actuating electrode. Two types of floating gate were fabricated; one is a top-floating gate ( Supplementary Fig. S1b ) and the other is a side-floating gate ( Supplementary Fig. S1c ) with an 80 nm Al 2 O 3 dielectric layer followed by 2 nm Ti/38 nm Au. These floating gates function as data storage capacitors for the non-volatile memory cell. Finally, the MEM cantilever, having an air-gap of 500 nm, was fabricated above the actuating electrode and the floating gate as shown in Supplementary Figure S1d . Finally, the device was lifted-off and dried in a critical point drier. Dose variation technique to produce the MEM cantilever To reduce the fabrication steps for making the suspended cantilever structures, we used the dose variation exposure technique, which controls the amount of dose precisely and develops selectively multi-layered resists [33] , [34] . Double layers of polymethylmethacrylate 950 K 4% were spin coated at 3,000 r.p.m. and baked for 5 min at 180 °C. Then, double layers of copolymer (MMA (8.5) MAA) ethyl lactate (EL) 10% were coated at the same speed and temperature, shown in Supplementary Figure S2a . Cantilever structures were exposed with varying dose conditions using EBL ( Supplementary Fig. S2b ). The colour bar indicates the dose levels of 170–450 μC cm −2 . The end of the pattern was slightly over-exposed with a dose of 190 μC cm −2 , so we can obtain a point contact structure between the end of the suspended cantilever and the floating gate beneath. The resists were developed for 20 min in a mixture of methyl isobutyl ketone and isopropanol in a ratio of 1:2. The exposed area with the dose of 170 μC cm −2 was developed only in the EL10 layer and the remaining polymethylmethacrylate resists acted as sacrificial layers for the suspended structure ( Supplementary Fig. S2c ). After development, the pattern was metalized with 1 nm Cr/200 nm Al/0.8 nm Cr. Cr was used to prevent oxidation of the Al layer and to reduce the residual stress in the cantilever ( Supplementary Fig. S2d ). Finally, the structure was lifted-off in acetone overnight and dried using a critical point drier ( Supplementary Fig. S2e ). Supplementary Figure S2f shows the field-emission scanning electron microscope images of a point contact structure that prevented any sticking problems for the MEMS device. Electrical characteristics of CNT-FET The devices were electrically characterized in air at room temperature using a drain-source bias of V ds =100 mV and various voltages on the Si substrate and cantilever. The transfer characteristics for a typical CNT-FET determined by a back gate sweep from −10 V to +10 V with V ds =100 mV are presented in Supplementary Figure S3a (side-floating gate type) and Supplementary Figure S3b (top-floating gate type). The devices show p-type behaviour with an on/off ratio of 10 4 –10 5 . The pull-in voltage ( V p ) of the cantilever was tested by increasing a positive voltage on the actuating electrode while keeping the cantilever grounded. Most of the devices showed a pull-in voltage, V p within the range of 14–18 V. Normally, the driving voltage ( V d ) applied to a MEMS cantilever is ∼ 1.2–1.4 times higher than the V p to assure stable mechanical contact [20] . For this reason, we applied a potential difference of 16 V (side-floating gate type, V p =14 V) and 24 V (top-floating gate type, V p =18 V) to each device. Mechanical resonance frequency and switching speed test The resonance frequency test was carried out by using the optical interferometer method [35] . The schematic of the measurement set up is shown in Supplementary Figure S4a . The ac signal was applied through the actuation electrode located under the suspended micro cantilever structure. The change of the reflected laser signal from the cantilever on mechanical resonance was detected by the high-speed photo receiver. Supplementary Figure S4b is the mechanical resonance measurement result of the microcantilever in our CNT-based MEM memory device. The mechanical resonance frequency of the cantilever was detected to be 8.5 MHz. The switching speed measurements were performed using a function generator (Yokogawa FG300), a high precision oscilloscope (Yokogawa DL1740 Digital Oscilloscope, Yokogawa), and an amplifier (NF HAS4101 High speed bipolar amplifier) in ambient atmosphere. Supplementary Figure S5a shows the schematic measurement set up. A square shape input signal with amplitude of 13 V was applied between the cantilever and actuation electrode and the output signal at the drain electrode was monitored with the oscilloscope. Note that for this experiment, a new three terminal micromechanical system, which has no floating gate was prepared so that we could measure the time at which contact was made between the cantilever and the drain electrode (taking the place of the floating gate). The dimension of the cantilever and the fabrication procedure is the same as for the floating-gate devices presented in the main paper. Supplementary Figures S5b and S5c show the switching speed measurement results of the switching motion and release motion respectively. Also, Supplementary Figures S5d and S5e show that the circuit delay times of our experimental setup for the switching signals are ca 35 ns. The time for switching on the device was found to be ca130 ns with a time of ca 145 ns to switch off. How to cite this article: Lee, S.W. A fast and low-power microelectromechanical system-based non-volatile memory device. Nat. Commun. 2:220 doi: 10.1038/ncomms1227 (2011).